A chronic model of arthritis supported by a strain-specific periarticular lymph node in BALB/c mice Current animal models of arthritis only partially reflect the complexity of rheumatoid arthritis and typically lack either chronicity or autoantibody formation. Here we describe a model that combines features of antigen-induced arthritis and collagen-induced arthritis, which can be efficiently induced in BALB/c and C57BL/6 mice. However, BALB/c mice generate significantly higher titres of anticollagen and anticitrullinated peptide antibodies, show a stronger progressive joint destruction, and in the chronic phase the disease spreads between joints. Concomitant to the observation of a more severe pathology, we discovered a previously undescribed small periarticular lymph node in close proximity to the knee joint of BALB/c mice, which acts as the primary draining lymph node for the synovial cavity. Our model more closely reflects the pathology of rheumatoid arthritis than classical models of arthritis and is hence particularly suitable for further studies of disease pathogenesis. Rheumatoid arthritis (RA) is a chronic inflammatory autoimmune disease characterized by a persistent synovitis that can lead to long-term joint damage, resulting in chronic pain, loss of function and disability [1] . The aetiology of RA comprises environmental, as well as genetic factors though the trigger for the onset of articular inflammation is still unknown. Most RA patients develop autoantibodies such as the rheumatoid factor or anticitrullinated peptide/protein antibodies (ACPA). The latter are highly specific for RA [2] , [3] and may be detected years before disease onset [4] , [5] . Moreover, the presence of ACPA is associated with a more severe joint destruction, the hallmark of RA [6] , [7] . About 50% of the risk for the development of RA has been attributed to genetic factors; however, most genomic regions associated with RA appear to be of low penetrance. The only genomic region that has emerged in all ethnic groups is the major histocompatibility complex (MHC) region and most prominently, the MHC class II gene cluster HLA-DRB1. The genetic association of RA to HLA-DRB1 alleles encoding the shared epitope is entirely confined to ACPA-positive RA as the shared epitope associates with the presence of antibodies directed against cyclic citrullinated peptides (anti-CCP antibodies), but not the presence of rheumatoid factor or RA as such [8] . In contrast, few mouse models of arthritis are associated with the development of ACPA. Mouse models of arthritis are indispensable tools for the investigation of cellular and molecular mechanisms underlying disease development; however, current models do not recapitulate a chronic autoimmune disease that spreads to the unaffected joints during disease progression. Similar to RA, most models are dependent on the genetic background of the animals; this hampers the use of gene-deficient mice as these are usually only available in the BALB/c or C57BL/6 background. The most commonly used mouse models are antigen-induced arthritis (AIA) and collagen-induced arthritis (CIA). AIA is induced by systemic immunization with an immunogenic antigen such as methylated BSA (mBSA) and subsequent intra-articular injection of mBSA into the knee joint. It has a strong inflammatory bias as shown by strong granulocyte infiltration and oedema formation in the acute phase of the disease (day 1–5 after induction) [9] . AIA reflects many symptoms of chronic RA, such as a strong synovitis with a dense infiltration of the synovial membrane by mononuclear cells and subsequent cartilage and bone erosion. Moreover, repeated inflammatory stimuli can induce the development of chronic arthritis. In CIA, systemic immunization with heterologous type II collagen (CII) in Freund’s complete adjuvant (CFA) leads to erosive arthritis in about 80% of the animals of susceptible mouse strains. CIA develops within ~3 weeks, but it is restricted to MHC class II subtypes I-A q , I-A r and H-2 q -bearing strains and has a remitting disease course [10] . Both models induce the formation of CII-specific antibodies although serum levels are higher in CIA. Yet, neither model develops the hallmark features of human chronic RA: the presence of ACPA and continuous spreading of disease, which usually starts from few joints. In order to mimic human joint-specific autoimmunity more closely we sought to add the CII-specific immunity of CIA to the chronic AIA model. We tested the combined antigen- and collagen-induced arthritis (ACIA) model in C57BL/6 and BALB/c mice, as both strains are commonly used for the generation and analysis of transgenic and knockout animals in biomedical research. Owing to genetic differences between BALB/c and C57BL/6 mice, such as different MHC haplotypes, these strains do respond differently in models of infection and autoimmunity. Whereas C57BL/6 mice develop only very weak arthritis in ACIA, BALB/c mice show a rapid onset of inflammation and higher values for common RA parameters, as shown by histological analysis and the development of ACPA, the most accurate prognostic marker of human RA. All the more, joint inflammation spreads to initially unaffected joints in the chronic phase of arthritis. The difference in disease development between BALB/c and C57BL/6 mice may in part pertain to the existence of a small periarticular lymph node (paLN) in untreated BALB/c but not in untreated C57BL/6 mice that acts as the primary draining lymph node for the knee joint. This previously undescribed lymph node in close proximity to the knee joint contributes to the local development of autoantibodies as observed by the formation of functional germinal centres (GCs) and the presence of antigen-specific plasma cells in this lymph node following arthritis induction. The ACIA model of chronic arthritis will be instrumental in further exploring the molecular and cellular mechanisms underlying chronic joint inflammation and in defining the role of autoreactive local follicular nodes in localized chronic diseases. ACIA induces chronic autoimmune arthritis in BALB/c mice BALB/c and C57BL/6 mice were immunized with mBSA in CFA and 1 week later with mBSA and bovine CII in Freund’s incomplete adjuvant. In addition, mice received Bordetella pertussis toxin (PTx) intraperitoneally at both time points to enhance the immune response. Arthritis was induced by a single injection of mBSA into the left knee-joint cavity ( Fig. 1a ). This combined AIA/CIA (ACIA) protocol induces a strong inflammation of the knee joint characterized by fibrinous exudates and an influx of neutrophils into the synovial cavity within the first 4 days after arthritis induction ( Fig. 1c ). After 4–7 days, fibrin exudation ceases and synovial hyperplasia with a massive infiltration of mononuclear cells can be observed. Eventually, arthritis passes into the chronic phase 3–4 weeks after induction. Chronic inflammation was characterized by dense clusters of lymphocyte infiltrates in the synovial and parasynovial tissue, chronic fibrosis and cartilage, as well as bone erosion ( Fig. 1c , right panel). The severity of chronic inflammation and joint destruction was evaluated by semiquantitative scoring of hematoxylin and eosin (HE)-stained paraffin sections of the left, that is, induced knee joint. The score for chronic inflammation reflects synovial hyperplasia, infiltration of the synovium by mononuclear cells and fibrosis. Joint destruction scores are based on pannus formation and cartilage and bone erosion. The histological analysis revealed no significant differences between BALB/c and C57BL/6 mice during the acute phase of inflammation; however, BALB/c mice showed significantly elevated scores for chronic arthritis compared with C57BL/6 animals. In particular, we observed joint destruction with massive bone erosion and calcification of cartilage tissue only in BALB/c but not in C57BL/6 mice ( Fig. 1b ). 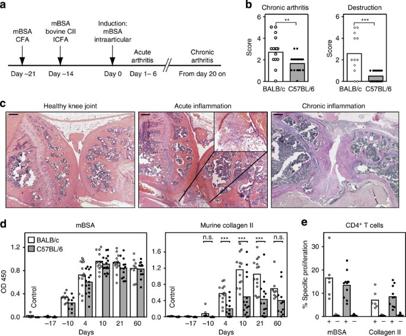Figure 1: ACIA leads to chronic autoimmune arthritis in BALB/c mice. (a) Time line of immunization procedure and development of arthritis. CFA, Freund’s complete adjuvant, ICFA, Freund’s incomplete adjuvant, mBSA, methylated bovine serum albumine, CII, bovine collagen type II. (b) Disease chronicity (left) and joint destruction (right) were assessed by scoring histology sections of BALB/c and C57BL/6 mice 5–8 weeks after arthritis induction. Statistics: Mann–Whitney-U-test,n=12–21, White bars indicate the mean value for BALB/c, grey bars for C57BL/6 samples. (c) HE-stained sections of paraffin-embedded knee joints from healthy (left) and arthritic BALB/c mice in the acute (middle) or chronic (right) inflammation phase. Black bars, 200 μm. (d) Arthritis-specific antibody production was higher in BALB/c than in C57BL/6 mice. Serum was tested at different time points in disease development for (auto)antibodies directed against the inducing agent mBSA and murine Collagen II using ELISA. Time points: healthy untreated, 4 days after first immunization (−17 days), 4 days after second immunization (−10 days), acute phase (4 days after induction), transition phase (10 days after induction), early chronic phase (3 weeks after induction) and late chronic phase (8–9 weeks after induction). White bars indicate the mean value for BALB/c, grey bars for C57BL/6 samples. Data is representative of two independent experiments with 8–15 animals per time point and group. Statistics: Mann–Whitney-U-test. (e) Generation of mBSA- and Collagen II-specific CD4+T cells by BALB/c and C57BL/6 mice in ACIA. Cells from the draining lymph nodes of immunized (+) or control (−) mice were stained with E-Fluor 670 and stimulated with mBSA or CII for 3 days. Cell proliferation was analysed by flow cytometry. Proliferating antigen-specific cells are indicated as percentages of CD4+lymphocytes. White bars indicate the mean value for BALB/c, grey bars for C57BL/6 samples. Data is representative of two independent experiments with 8–15 animals per group. Statistics: Mann–Whitney-U-test (n.s., not significant, OD, optical density, *P<0.05, **P<0.01, ***P<0.001). Figure 1: ACIA leads to chronic autoimmune arthritis in BALB/c mice. ( a ) Time line of immunization procedure and development of arthritis. CFA, Freund’s complete adjuvant, ICFA, Freund’s incomplete adjuvant, mBSA, methylated bovine serum albumine, CII, bovine collagen type II. ( b ) Disease chronicity (left) and joint destruction (right) were assessed by scoring histology sections of BALB/c and C57BL/6 mice 5–8 weeks after arthritis induction. Statistics: Mann–Whitney- U -test, n =12–21, White bars indicate the mean value for BALB/c, grey bars for C57BL/6 samples. ( c ) HE-stained sections of paraffin-embedded knee joints from healthy (left) and arthritic BALB/c mice in the acute (middle) or chronic (right) inflammation phase. Black bars, 200 μm. ( d ) Arthritis-specific antibody production was higher in BALB/c than in C57BL/6 mice. Serum was tested at different time points in disease development for (auto)antibodies directed against the inducing agent mBSA and murine Collagen II using ELISA. Time points: healthy untreated, 4 days after first immunization (−17 days), 4 days after second immunization (−10 days), acute phase (4 days after induction), transition phase (10 days after induction), early chronic phase (3 weeks after induction) and late chronic phase (8–9 weeks after induction). White bars indicate the mean value for BALB/c, grey bars for C57BL/6 samples. Data is representative of two independent experiments with 8–15 animals per time point and group. Statistics: Mann–Whitney- U -test. ( e ) Generation of mBSA- and Collagen II-specific CD4 + T cells by BALB/c and C57BL/6 mice in ACIA. Cells from the draining lymph nodes of immunized (+) or control (−) mice were stained with E-Fluor 670 and stimulated with mBSA or CII for 3 days. Cell proliferation was analysed by flow cytometry. Proliferating antigen-specific cells are indicated as percentages of CD4 + lymphocytes. White bars indicate the mean value for BALB/c, grey bars for C57BL/6 samples. Data is representative of two independent experiments with 8–15 animals per group. Statistics: Mann–Whitney- U -test (n.s., not significant, OD, optical density, * P <0.05, ** P <0.01, *** P <0.001). Full size image Next, we compared both mouse strains for the development of antibodies to the arthritis-inducing antigens mBSA and CII ( Fig. 1d ). Mice were bled at several time points before and after arthritis induction and antibody levels determined by enzyme-linked immunosorbent assay (ELISA). Low levels of IgG specific for the main antigen mBSA could be detected shortly after the second immunization. In both strains antibody titres reached peak levels around day 10 following arthritis induction ( Fig. 1d , left panel). This accords with the observation that AIA development is comparable in BALB/c and C57BL/6 mice 9 . As mice have been additionally immunized with heterologous CII from bovine trachea to break tolerance and promote an autoimmune response, we tested for the generation of autoreactive antibodies directed against murine CII. Both strains develop CII-specific IgG with a similar kinetic profile ( Fig. 1d , right panel). However, in the acute and early chronic phase, anti-CII antibody titres were significantly higher in BALB/c mice than in C57BL/6 mice, indicating a stronger humoral response of BALB/c mice in the combined ACIA model. Generation of antigen-specific T-cell responses in ACIA CD4 + T cells are known to have a crucial role in arthritis [11] . Therefore, we tested whether BALB/c and C57BL/6 mice differ in their capacity to generate antigen-specific, that is, mBSA- and CII-specific, T cells in the new ACIA model. Figure 1e shows the proliferative response of T cells isolated from the popliteal and inguinal lymph nodes of mice immunized with mBSA and CII and healthy control animals. T-cell proliferation in response to mBSA or CII does not differ between immunized C57BL/6 and BALB/c mice; hence, the generation of antigen-specific T cells is probably not responsible for the differences in joint destruction and ACPA titres observed between the two mouse strains in ACIA. BALB/c mice develop a paLN A histological analysis of the chronically inflamed knees with their surrounding tissue revealed the existence of a lymph node-like structure in close proximity to knee joints in BALB/c mice ( Fig. 2a ) that was not detectable in C57BL/6 mice. These periarticular structures were smaller in size than the popliteal lymph node and also present in healthy BALB/c animals, albeit at a smaller size ( Fig. 2c ). We next asked whether these structures are fully accessible to lymphocytes via the circulation. To test this, we transferred biotin-labelled splenocytes intravenously into arthritic animals and analysed the spleens and periarticular structures 18 h later for the presence of the transferred cells. Splenocytes were able to access not only the spleen but also the periarticular nodes, indicating that these follicles are fully functional lymph nodes ( Fig. 2d ). Finally, we characterized these structures for typical features of secondary lymphoid organs such as T/B compartmentalization and GC formation. Double staining of paraffin sections for T cells (CD3, red) and B cells (B220, blue) revealed a clear T-cell—B-cell segregation both in naive and arthritic animals ( Fig. 2e ). Both groups of mice showed networks of follicular dendritic cells (FDCs) within the B cell zones (FDC-M2, blue), lymphatic vessels (LYVE-1, blue) and high endothelial venules (PNAd, blue) in these periarticular structures ( Fig. 2e ). In contrast, GC formation could only be detected after arthritis induction, by staining with peanut agglutinin (PNA) and for Ki67, a marker for proliferating cells. The number of proliferating cells increased from day 4 on and both GCs and proliferative activity persisted until the end of the period examined. Given the full functionality of a regular lymph node we term the newly discovered periarticular structures paLN. 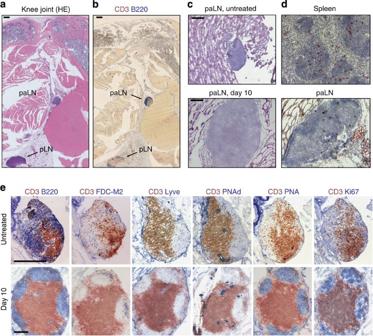Figure 2: BALB/c mice develop an additional paLN in close vicinity to the knee joint. (a) Section of paraffin-embedded hind leg from BALB/c mouse in the early chronic phase of RA with hematoxylin eosin staining. Arrows: periarticular lymph node (paLN) close to the knee joint and popliteal lymph node (pLN) embedded in fat tissue. Black bars, 400 μm. (b) paLN and popliteal lymph node stained for B cells (B220, blue) and T cells (CD3, red). (c) HE staining of cryosections of paLN in healthy untreated BALB/c mice (top) and 10 days after induction of arthritis (bottom). Black bars, 200 μm. (d) paLNs are connected to the vasculature. Biotinylated splenocytes were injected intravenously into arthritic mice. Eighteen hours after transfer, biotinylated cells (in red) could be detected in the spleen (top) and the paLN (bottom). Magnification X40. (e) paLNs are fully functional and develop GCs following arthritis induction. Characterization of the microarchitecture of the paLN from healthy and arthritic BALB/c mice: T cells were stained with peroxidase-labelled anti-CD3 antibody (in red) and several other lymph node and activation markers (in blue). FDC-M2 is a marker for FDCs, Lyve for lymphatic vessels, PNAd for high endothelial venules, PNA for GCs and Ki67 for proliferating cells. Only after arthritis induction, GCs are formed that harbour proliferating cells. The tissue sections represent two independent experiments with four animals per time point. Magnification: X40 for lymph nodes isolated 10 days after induction of arthritis and X100 for lymph nodes from healthy untreated mice. Black bars, 200 μm. Figure 2: BALB/c mice develop an additional paLN in close vicinity to the knee joint. ( a ) Section of paraffin-embedded hind leg from BALB/c mouse in the early chronic phase of RA with hematoxylin eosin staining. Arrows: periarticular lymph node (paLN) close to the knee joint and popliteal lymph node (pLN) embedded in fat tissue. Black bars, 400 μm. ( b ) paLN and popliteal lymph node stained for B cells (B220, blue) and T cells (CD3, red). ( c ) HE staining of cryosections of paLN in healthy untreated BALB/c mice (top) and 10 days after induction of arthritis (bottom). Black bars, 200 μm. ( d ) paLNs are connected to the vasculature. Biotinylated splenocytes were injected intravenously into arthritic mice. Eighteen hours after transfer, biotinylated cells (in red) could be detected in the spleen (top) and the paLN (bottom). Magnification X40. ( e ) paLNs are fully functional and develop GCs following arthritis induction. Characterization of the microarchitecture of the paLN from healthy and arthritic BALB/c mice: T cells were stained with peroxidase-labelled anti-CD3 antibody (in red) and several other lymph node and activation markers (in blue). FDC-M2 is a marker for FDCs, Lyve for lymphatic vessels, PNAd for high endothelial venules, PNA for GCs and Ki67 for proliferating cells. Only after arthritis induction, GCs are formed that harbour proliferating cells. The tissue sections represent two independent experiments with four animals per time point. Magnification: X40 for lymph nodes isolated 10 days after induction of arthritis and X100 for lymph nodes from healthy untreated mice. Black bars, 200 μm. Full size image The paLN drains the synovial cavity Secondary lymphoid organs have an essential role in tissue immune surveillance. Each lymph node drains and controls a specific part of the body. To find out whether the synovial cavity is drained by the periarticular or popliteal lymph node in BALB/c mice, we transferred biotinylated splenocytes directly into the knee joint of healthy animals. Mice were killed 18 or 24 h after transfer and cryosections of the periarticular, popliteal and inguinal lymph nodes were stained for immigrated splenocytes. Within 18 h, a large number of cells had migrated into the paLN, whereas no cells could be detected in the popliteal or inguinal lymph nodes ( Fig. 3 , top). However, after 24 h a very limited number of transferred splenocytes were found scattered in the popliteal lymph node ( Fig. 3 , bottom, black arrows). Thus, our data strongly implies that the paLN is the primary draining lymph node for the knee joint cavity. 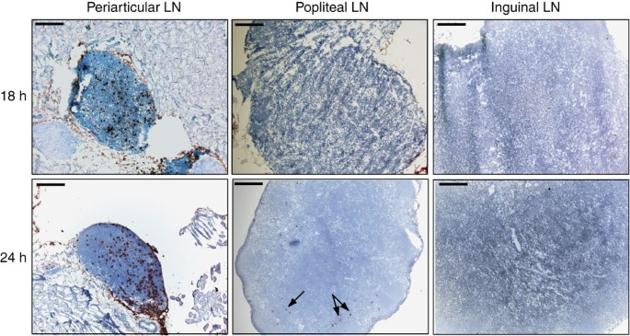Figure 3: The paLN acts as the primary draining lymph node for the synovial cavity. Biotinylated splenocytes were injected intra-articularly into the knee joint of healthy BALB/c mice. Periarticular (left), popliteal (middle) or inguinal (right) lymph nodes were prepared 18 h (top) or 24 h (bottom) after injection. Splenocytes were visualized in red by staining with peroxidase-labelled streptavidin and AEC; counterstaining with hematoxylin is shown in blue. Sections are representative for three independent experiments. Black bars, 200 μm. Figure 3: The paLN acts as the primary draining lymph node for the synovial cavity. Biotinylated splenocytes were injected intra-articularly into the knee joint of healthy BALB/c mice. Periarticular (left), popliteal (middle) or inguinal (right) lymph nodes were prepared 18 h (top) or 24 h (bottom) after injection. Splenocytes were visualized in red by staining with peroxidase-labelled streptavidin and AEC; counterstaining with hematoxylin is shown in blue. Sections are representative for three independent experiments. Black bars, 200 μm. Full size image Antigen-specific immune responses in the paLN Having shown that active GCs are formed in the paLN after the onset of arthritis, we wanted to further explore their involvement in the autoimmune response. In arthritic mice we were able to detect cells specific for mBSA in the paLN ( Fig. 4a ). All the more, we could detect CD138-positive plasma cells that co-localize with the mBSA-specific cells within the GCs of the paLN ( Fig. 4b ). Hence, within these GCs B cells can differentiate into mature plasma cells expressing antibodies directed against a local (auto)antigen. When comparing the paLN directly with the popliteal lymph node it became obvious that only few single plasma cells were present in the popliteal lymph node, whereas the paLN harboured large areas of CD138 + plasma cells within the B cell zones. 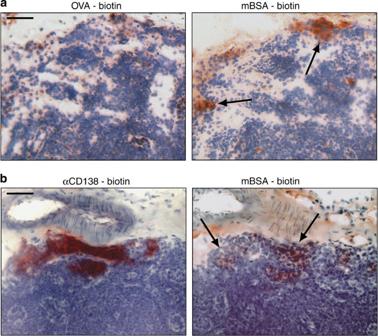Figure 4: Generation of antigen-specific plasma cells in the GCs of the paLN. Consecutive cryosections of the paLN from BALB/c mice with chronic arthritis were stained in red for binding of the irrelevant protein ovalbumin (a, left panel) or biotinylated mBSA (a, right panel). The paLN was stained for plasma cells with a biotinylated anti-CD138 antibody (b, left panel) or biotinylated mBSA (b, right). Sections are representative for three independent experiments. Magnification X200. Figure 4: Generation of antigen-specific plasma cells in the GCs of the paLN. Consecutive cryosections of the paLN from BALB/c mice with chronic arthritis were stained in red for binding of the irrelevant protein ovalbumin ( a , left panel) or biotinylated mBSA ( a , right panel). The paLN was stained for plasma cells with a biotinylated anti-CD138 antibody ( b , left panel) or biotinylated mBSA ( b , right). Sections are representative for three independent experiments. Magnification X200. Full size image Development of antibodies to citrullinated antigens in ACIA Current models of arthritis usually fail to recapitulate the formation of ACPA. These autoantibodies, however, are the most important biomarker for RA development in clinical practise. The best-known triggers for antibodies to citrullinated peptides are filaggrin, CII, α-enolase, fibrin(ogen) and vimentin. Antibodies directed against a mutated citrullinated isoform of vimentin (MCV) can also be detected in the synovial fluid of RA patients. These anti-MCV antibodies seem to have a higher sensitivity for RA compared with antibodies against artificial CCPs [12] . We were able to detect both, anti-CCP and anti-MCV antibodies in the serum of BALB/c and C57BL/6 mice in the ACIA model ( Fig. 5 ). Antibodies to CCP were already detectable at day −10 before arthritis induction. Serum titres of anti-CCP antibodies that are significantly higher in BALB/c than in C57BL/6 mice increased until day 10 after immunization, then they reached a plateau ( Fig. 5a ). In contrast, elevated titres of anti-MCV autoantibodies become apparent shortly after arthritis induction (day 4). Similar to anti-CCP, antibody titres reach a maximum at day 10 after arthritis induction. Compared with BALB/c mice C57BL/6 animals are inefficient in the induction of anti-MCV antibodies ( Fig. 5b ). The high titres of ACPA in ACIA led us to investigate whether PTx, which is included in the classical immunization scheme of AIA but not CIA [9] , [13] , [14] , has an impact on ACPA formation. Similar to the observation that PTx boosts the antibody-response to mBSA in AIA, we observed significantly higher levels of ACPA in BALB/c mice receiving PTx compared with BALB/c mice receiving PBS ( Fig. 5c ). Still, the generation of ACPA does not depend on PTx as ACPA formation is delayed but robust also in the absence of PTx as adjuvant. 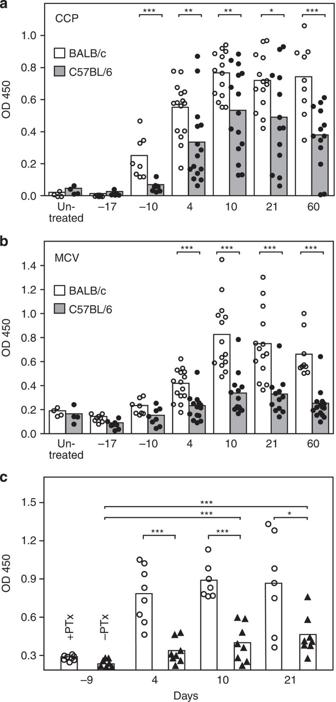Figure 5: BALB/c mice develop high titres of ACPA after arthritis induction. Serum of untreated, immunized or arthritic BALB/C and C57BL/6 mice was tested with ELISA for antibodies against ACPA: CCP (a) and MCV (b). Time points: healthy untreated, 4 days after first immunization (−17 days), 4 days after second immunization (−10 days), acute phase (4 days after induction), transition phase (10 days after induction), early chronic phase (3 weeks after induction), and late chronic phase (8–9 weeks after induction). White bars indicate mean values for BALB/c, grey bars for C57BL/6 samples. Data is representative of two independent experiments with 8–15 animals per time point and group. (c) The presence of pertussis toxin during immunization influences ACPA levels. BALB/c mice were immunized according to the ACIA scheme with or without PTx and levels of anti-CCP antibodies compared at different disease stages. Time points: 4 days after second immunization (−9 days), acute phase (4 days after induction), transition phase (10 days after induction), early chronic phase (3 weeks after induction). Mice were immunized according to the ACIA scheme with either PTx (circles) or PBS instead of PTx (triangles). Statistics: Mann–Whitney-U-test (n.s.: not significant, *P<0.05, **P<0.01, ***P<0.001). Figure 5: BALB/c mice develop high titres of ACPA after arthritis induction. Serum of untreated, immunized or arthritic BALB/C and C57BL/6 mice was tested with ELISA for antibodies against ACPA: CCP ( a ) and MCV ( b ). Time points: healthy untreated, 4 days after first immunization (−17 days), 4 days after second immunization (−10 days), acute phase (4 days after induction), transition phase (10 days after induction), early chronic phase (3 weeks after induction), and late chronic phase (8–9 weeks after induction). White bars indicate mean values for BALB/c, grey bars for C57BL/6 samples. Data is representative of two independent experiments with 8–15 animals per time point and group. ( c ) The presence of pertussis toxin during immunization influences ACPA levels. BALB/c mice were immunized according to the ACIA scheme with or without PTx and levels of anti-CCP antibodies compared at different disease stages. Time points: 4 days after second immunization (−9 days), acute phase (4 days after induction), transition phase (10 days after induction), early chronic phase (3 weeks after induction). Mice were immunized according to the ACIA scheme with either PTx (circles) or PBS instead of PTx (triangles). Statistics: Mann–Whitney- U -test (n.s. : not significant, * P <0.05, ** P <0.01, *** P <0.001). Full size image Induction of systemic joint inflammation in chronic ACIA Early RA is predominantly a local, articular matter. Later, the inflammation disseminates to other joints and may eventually become systemic. To test whether the ACIA model leads to systemic joint inflammation in the chronic phase, we analysed the synovial fluid of the knee joint cavities in the acute phase 4 days and 5–8 weeks after induction of arthritis ( Fig. 6a ). We compared the induced (left) with the non-induced (right) knee joints and found, as expected, in the synovial fluid from the left knee joints a manifold increase in the number of cells in the acute phase with high numbers of neutrophils (black arrows), macrophages (red arrows) and mononuclear cells. However, we did not observe cellular infiltration in synovial fluid from the non-induced knee joints during the acute phase of the disease ( Fig. 6b ). In the chronic phase, 8 weeks after arthritis induction, we observed a decrease in the number of infiltrating cells compared with the acute phase, but the number of cells present in the synovial fluid was still elevated. In the chronic phase the infiltrate was mainly composed of mononuclear and fibroblast-like cells. Interestingly, 8 weeks after local induction of arthritis in the left knee joint, we observed also high numbers of infiltrating cells in the synovial fluid of the non-induced knee joint ( Fig. 6b ). The histological analysis showed no signs of inflammation in the non-induced knee joints on day 4 ( Fig. 6c ); however, 4 weeks after induction we observed typical signs of chronic inflammation such as cellular infiltration, hyperplasia of the synovial membrane and fibrosis. Scoring of the sections confirmed spreading of inflammation to non-induced knee joints in the chronic phase of ACIA ( Fig. 6d ). 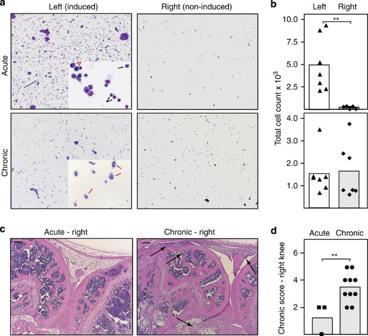Figure 6: Spreading of arthritis to non-induced joints in chronic ACIA. (a) Cytospins with May-Gruenwald-Giemsa staining of the synovial fluid of the left (induced) or right (non-induced) knee joint in the acute (4 days after induction) and chronic (5–8 weeks after induction) inflammation phase. Magnification X50 and X400. (b) Quantification of cells in the SF in the acute (top) and chronic phase (bottom). In the chronic phase a comparable number of cells is found in the synovial fluid of the induced and non-induced knee joints; the inflammation spreads to other joints. (c) HE staining of paraffin sections of the non-induced right knee joints in the acute (left) or chronic (right) phase of arthritis. Arrows indicate hallmarks of chronic inflammation: cell infiltrations, the hyperplastic synovial membrane and fibrosis. Black bars, 200 μm. (d) Scoring of histology sections for chronic inflammation in the non-induced (right) knee joint of BALB/c mice in the acute phase (day 4, squares) and chronic phase 5–8 weeks after induction of arthritis (circles). Scoring statistics: Mann–Whitney-U-test (n.s.: not significant, *P<0.05, **P<0.01, ***P<0.001). Figure 6: Spreading of arthritis to non-induced joints in chronic ACIA. ( a ) Cytospins with May-Gruenwald-Giemsa staining of the synovial fluid of the left (induced) or right (non-induced) knee joint in the acute (4 days after induction) and chronic (5–8 weeks after induction) inflammation phase. Magnification X50 and X400. ( b ) Quantification of cells in the SF in the acute (top) and chronic phase (bottom). In the chronic phase a comparable number of cells is found in the synovial fluid of the induced and non-induced knee joints; the inflammation spreads to other joints. ( c ) HE staining of paraffin sections of the non-induced right knee joints in the acute (left) or chronic (right) phase of arthritis. Arrows indicate hallmarks of chronic inflammation: cell infiltrations, the hyperplastic synovial membrane and fibrosis. Black bars, 200 μm. ( d ) Scoring of histology sections for chronic inflammation in the non-induced (right) knee joint of BALB/c mice in the acute phase (day 4, squares) and chronic phase 5–8 weeks after induction of arthritis (circles). Scoring statistics: Mann–Whitney- U -test (n.s. : not significant, * P <0.05, ** P <0.01, *** P <0.001). Full size image Current mouse models of RA have limitations as they are lacking the complexity of the human disease. Most models fail to develop an autoantigen-driven chronic course of the disease, or lack the formation of RA-specific autoantibodies like ACPA, and they are restricted to few susceptible strains which are not commonly used in immunological research [15] , [16] . To better mimic the combination of autoantibody production and disease chronicity as observed in RA, we developed a novel mouse model of arthritis by combining classical antigen-induced arthritis (AIA) and CIA. The objective of this strategy was to break tolerance against endogenous collagen by inducing a strong local inflammation with the help of the potent immunogen mBSA. We were particularly interested in a model applicable to mouse strains such as BALB/c and C57BL/6, of which large numbers of genetically modified variants allow for a detailed analysis of the molecular mechanisms underlying the disease. Similar to RA, susceptibility of mice to arthritis has been associated with the expression of certain MHC class II molecules. AIA can be induced in different genetic backgrounds including C57BL/6 and BALB/c strains harbouring the MHC haplotypes H2-K b /I-A b and H2-K d /I-A d , respectively [9] . In contrast, CIA using bovine CII as antigen, is largely restricted to mice bearing the MHC haplotypes H2-K q /I-A q (for example, DBA/1 mice) or H2-K r /I-A r (for example, B10.RIII mice) [10] , [17] . Nevertheless, an increased amount of mycobacterial components or the use of chicken CII has been reported to induce a mild form of CIA also in C57BL/6 mice [18] , [19] . As for the BALB/c mouse strain, the repeated subcutaneous application of collagen emulsified in CFA induces arthritis-like symptoms in 60–80% of the treated mice when coadministered with a non-self protein such as ovalbumin [20] . However, the histopathological scores were low in that model and the induction of autoimmune reactions such as ACPA formation or spreading of the disease has not been shown. In ACIA, both BALB/c and C57BL/6 mice develop an acute inflammation of the knee joint including synovial hyperplasia and comparable titres of antibodies against the artificial antigen mBSA. However, only BALB/c mice develop chronic arthritis with joint destruction, bone erosion and calcification of cartilage tissue, which eventually spreads to other joints and turns systemic. The difference in the outcome of ACIA in the two mouse strains is most likely caused by a combination of factors including the genetic background, the local immunological environment and the generation of autoreactive antibodies. High titres of anti-CII antibodies in the serum of BALB/c but not C57BL/6 mice most likely contribute to the strong inflammatory response (and cartilage degradation) and thus promote disease chronicity. CII antibodies are found in the serum and synovial fluid of the majority of RA patients [21] , [22] . There are two mechanisms by which CII antibodies mediate joint inflammation in CIA. Firstly, they are reported to have a crucial role in the induction of inflammation by the formation of IgG immune complexes that crosslink Fc-receptors [23] , [24] . In addition, CII autoantibodies mediate joint inflammation in CIA by activating the complement system [25] . The ACIA model also induces a robust ACPA response that is enhanced by the adjuvant PTx. Citrullination is a post-translational modification, which occurs in inflammatory environments like the inflamed synovium of RA patients [26] . In dying cells, peptidyl deiminases become activated, convert peptidylarginine residues of cartilage extracellular matrix to peptidylcitrulline and thus give rise to neoantigens [27] . Seventy to eighty percent of RA patients are ACPA positive; the occurrence of ACPA is highly specific and currently the clinical marker with the highest prognostic value that can be detected even years before the onset of the disease [2] , [4] , [28] , [29] , [30] . Recent studies indicate that ACPA-positive RA results in a more severe disease pathology such as erosive cartilage degradation as compared with ACPA-negative disease (reviewed in refs 31 , 32 , 33 ). ACPA-positive RA shows a strong correlation to the major genetic risk factor, alleles of HLA-DRB1 encoding the shared epitope [34] , [35] . Interestingly, alleles encoding the shared epitope do not associate with RA as such but with anti-CCP + RA and disease progression is more severe in RA patients with both anti-CCP antibodies and shared epitope alleles [7] , [8] . Accordingly, some data suggest that ACPA are active pathogenic components of the RA autoimmune response as they form immune complexes with citrullinated antigens, activate the complement system and, thus, increase the production of proinflammatory cytokines and the recruitment of inflammatory cells [27] , [36] , [37] . Similar to the situation described in RA patients, autoantibody responses of mice in CIA successively expand to multiple epitopes with progression of the disease, this creation of neoantigens is referred to as epitope spreading [38] . In our study, two different assays for the detection of ACPA were compared: the CCP ELISA, where short CCPs serve as autoantigens and the MCV ELISA where the coated antigen is mutated and citrullinated vimentin, such as it is present in the inflamed synovium [12] . The MCV test was found to be more sensitive and to be correlating with the disease activity score in RA [39] , [40] . In addition, the MCV test was suggested to be used for monitoring the effect of infliximab therapy [41] . In the ACIA model, both assays yielded the same results, that is, a significantly stronger and more protracted ACPA response in arthritic BALB/c mice than in C57BL/6 mice. The high titre of anti-CII and anti-ACPA autoantibodies in arthritic BALB/c mice most likely contributed to the severe joint damage observed in the BALB/c mouse strain and the different outcome of our model in C57BL/6 mice. This finding reflects the situation in humans: ACPA-positive RA patients suffer from a more severe arthritis than patients without these autoantibodies [42] . There is increasing evidence that not only the draining lymph nodes of the affected joints but also ectopic lymphoid tissue that can be formed in or close to the synovium contributes to the production of ACPA and may enhance arthritis [43] , [44] . In a modified, strongly inflammatory model of AIA C57BL/6 mice developed after 3–6 months ectopic lymph node-like structures within the inflamed synovial tissue or between synovial and connective muscle tissue beneath the knee joint [45] . However, we found no evidence of lymphoid neogenesis in the ACIA model. Instead we discovered a previously undescribed lymph node in close proximity to the knee joint, which we named ’periarticular‘ lymph node (paLN), in mice of the BALB/c strain that could not be detected in C57BL/6 mice. One might speculate that in C57BL/6 mice rudimentary lymph node anlagen are present, which under normal conditions do not develop into fully functional lymph nodes. This paLN was the primary draining lymph node for the knee joint in BALB/c mice and clearly distinguishable from the popliteal lymph node. In case of an ongoing synovial inflammation, the paLN increased substantially in size by hosting a large number of activated lymphocytes. Once ACIA was established, we could detect GCs and mBSA-specific plasma cells within this paLN. We were not able to use the same experimental approach as for mBSA to identify CII-specific plasma cells on tissue sections due to the limited solubility and unspecific binding of CII. Our findings underline the presumable importance of local draining lymph nodes for the outcome of the ACIA arthritis model. This is consistent with observations in the K/BxN mouse model where the transgenic mice develop spontaneously arthritis-like symptoms [46] , [47] . In that model, the autoimmune B-cell responses are focused specifically in the local draining (distal) lymph nodes. All the more, removal of these lymph nodes resulted in a decreased B-cell response and autoantibody production, as well as a dramatic attenuation of arthritis [46] . The different levels of autoantibody formation in BALB/c and C57BL/6 mice may also indicate a role for the MHC and different affinities of autoantigen presentation. This aspect, however, was beyond the scope of our study. In summary, one might speculate that both genetic differences and the pre-existence of a paLN in BALB/c mice contribute to the different development of full chronic inflammation in both mouse strains. We assume that the rapid development of chronic, destructive arthritis in BALB/c mice using the ACIA model is based both on genetic and morphologic preconditions. The presence of local lymphoid tissues supporting ongoing autoimmune reactions may have a pivotal role for the progression of an acute local inflammatory process into a systemic autoimmune disorder. Thus, the absence of a paLN in C57BL/6 mice and a less-efficient MHC presentation of (auto)antigens could be the reason why their overall autoimmune responses in the ACIA model were weaker than those of BALB/c animals. Hence, the ACIA model might be particularly beneficial in studying site-specific autoimmune reactions. In BALB/c mice, the ACIA model leads to a profound synovitis with cartilage and bone erosion that spreads to other joints. Moreover, it is characterized by an efficient and rapid formation of autoantibodies directed against ACPA and CII. To our knowledge the ACIA model reflects more features of the pathology of RA than classical models of arthritis and is hence particularly suited to further study RA pathogenesis and to develop innovative therapeutic strategies. Mice Female BALB/c and C57BL/6 mice were purchased from Charles River Deutschland (Sulzfeld, Germany). Mice were used at 10–14 weeks of age. All animal studies were performed according to institutional and state guidelines, under specific pathogen-free conditions. AIA/CIA combined model Mice were immunized by subcutaneous injection of 100 μg mBSA (Sigma-Aldrich, Schnelldorf, Germany) in 50 μl of PBS emulsified with 50 μl of CFA (Sigma-Aldrich) at day –21. One week later, mice were immunized with 50 μg mBSA, 100 μg bovine collagen type II (mdbioproducts, Zurich, Switzerland) in 50 μl PBS emulsified with 50 μl Freund’s incomplete adjuvant (IFA, Sigma-Aldrich) subcutaneously. In parallel to each immunization step, 200 ng of Bordetella pertussis toxin (PTx, Calbiochem, La Jolla, CA, USA) were given intraperitoneally. Induction of arthritis was achieved by intra-articular injection of 50 μg mBSA dissolved in 20 μl of PBS into the left knee-joint cavity. Animals were analysed at various time points (4 days, 10 days, 3 weeks and 8 weeks after arthritis induction) reflecting different stages of the disease. Immunohistochemical analysis Animals were killed and both knee joints were fixed in 4% buffered formaldehyde, decalcified with EDTA, and embedded in paraffin. Serial sections (4–5 μm thick) were cut and stained with HE for microscopic evaluation. Scoring of the knee sections was performed in a blinded manner with examination of four sections per knee joint. A three parameter scoring system was used, where individual scores sum up: acute score (exudate 1–3 points, granulocytes infiltrating the synovial membrane 1–3 points and fibrin exudates+1 point), chronic score (synovial hyperplasia 1–3 points, mononuclear cells infiltrating the synovial membrane 1–3 points and fibrosis 1–3 points), cartilage and bone destruction (1–3 points). Alternatively to paraffin embedding knee tissue was cryopreserved: thigh and shank were removed and the remaining tissue was embedded in TissueTek O.C.T. compound (Sakura Finetek, Zoeterwoude, The Netherlands) and snap frozen in dry ice. The specimens were cut into 6–8 μm thick sections using a microtome, dried and dehydrated with ice-cold acetone. For immunohistochemistry, paraffin sections were deparaffinized and unmasked by heat; cryosections were rehydrated in Tris buffer. For staining, the following primary antibodies were used: anti-CD3ε (goat, Santa Cruz Biotechnology, Santa Cruz, CA), anti-CD45R/B220 (rat biotinylated, Biolegend Europe, Uithoorn, The Netherlands), anti-CD138 (rat biotinylated, Caltag-Invitrogen, Karlsruhe, Germany), anti-Ki67 (rat, DAKO, Hamburg, Germany), anti-PNAd/ anti-CD62L (BD Biosciences, Heidelberg, Germany), anti-FDC-M2 (rat biotinylated, Immunokontact, AMS Biotechnology, Oxfordshire, GB) anti-PNA (peanut lectin biotinylated, Sigma-Aldrich), anti-Lyve-1 (rabbit, Upstate Biotechnology, Lake Placid, NY). For detection biotinylated donkey anti-goat, donkey anti-rat or Peroxidase-coupled donkey anti-goat antibodies were added, followed by streptavidin-conjugated alkaline phosphatase (all from JacksonImmunoResearch, Newmarket, UK). Enzyme reactions were developed with AEC+Substrate Kit (DAKO) or Fast Blue substrate (Sigma-Aldrich). Isolation and labelling of splenocytes Splenocytes of wild-type mice were prepared and depleted of erythrocytes by treatment with red blood cell lysis buffer (150 mM NH 4 Cl, 10 mM KHCO 3 , 0.1 mM Na 2 -EDTA at pH 7.2). Splenocytes were washed with sterile PBS, biotinylated with Biotin N-succinimidyl ester (Sigma-Aldrich), and injected i.v. into the tail vein or intra-articularly into the knee joint. Transferred cells were stained on cryosections from spleen or lymph nodes of recipient mice with streptavidin-conjugated alkaline phosphatase as described above. T-cell proliferation Single-cell suspensions were prepared from inguinal lymph nodes 5 days after the second immunization. As controls, cells from the inguinal lymph nodes of age-matched untreated BALB/c mice were used. Lymph node cells were washed with PBS and stained with E-Fluor 670 to track cell proliferation. Cells were resuspended in RPMI 1640 medium supplemented with 10% heat-inactivated fetal calf serum, penicillin and streptomycin and 50 μM β-mercaptoethanol. Cells were cultured in 96-well plates (5 × 10 6 cells per well) in the presence of 25 μg ml −1 mBSA (Sigma-Aldrich) or 75 μg ml −1 bovine CII (Chondrex Inc., Redmond, WA, USA) for 3 days at 37 °C, in a 5% CO 2 atmosphere. Cells were then harvested, washed with FACS buffer, stained with a CD4 antibody (CD4-FITC, clone GK 1.5, Biolegend) and 7-AAD (BD Pharmingen) to exclude dead cells and analysed by flow cytometry for cell division. Immunoglobulin production and ELISA Analysis of antigen-specific IgG titres in serum was performed with capture ELISA. To measure mBSA-specific IgG Immunosorp microtiter plates (Nunc, Langenselbold, Germany) were coated with 2 μg per well mBSA in PBS. Bound serum antibodies were detected using horseradish peroxidase-conjugated rabbit anti-mouse serum (Southern Biotech, Eeling, Germany). Murine Collagen type II-specific antibodies were measured using the mouse IgG anti-Mouse Collagen Type II ELISA (mdbiosciences, Egg b. Zürich Switzerland). Antibody titres to CCPs were measured using Immunoscan CCPlus plates (Euro-Diagnostica, Malmo, Sweden) but replacing the detection solution with rabbit anti-mouse serum. No unspecific binding of the exchanged detection serum was observed. The Anti-MCV ELISA (Orgentec Diagnostica, Mainz, Germany) was used for the detection of MCV-specific antibodies. Synovial lavage Knee cavities were surgically opened and synovial lavage was obtained by sequential flushing of the joint cavity. Cytospin preparations were stained with May-Gruenwald-Giemsa to determine the cellular composition of the lavage fluid. Statistics Results are expressed as arithmetic means±s.e.m. All statistical analyses were performed using Prism 5.0 (GraphPad Software) and the non-parametric Mann–Whitney- U -test. Statistical differences with a probability of P <0.05 are indicated with *, P <0.01 with ** and P <0.001 with ***. How to cite this article: Baddack, U. et al . A chronic model of arthritis supported by a strain-specific periarticular lymph node in BALB/c mice. Nat. Commun. 4:1644 doi: 10.1038/ncomms2625 (2013).